Oestrogen signalling in white adipose progenitor cells inhibits differentiation into brown adipose and smooth muscle cells Oestrogen, often via oestrogen receptor alpha (ERα) signalling, regulates metabolic physiology, highlighted by post-menopausal temperature dysregulation (hot flashes), glucose intolerance, increased appetite and reduced metabolic rate. Here we show that ERα signalling has a role in adipose lineage specification in mice. ERα regulates adipose progenitor identity and potency, promoting white adipogenic lineage commitment. White adipose progenitors lacking ERα reprogramme and enter into smooth muscle and brown adipogenic fates. Mechanistic studies highlight a TGFβ programme involved in progenitor reprogramming downstream of ERα signalling. The observed reprogramming has profound metabolic outcomes; both female and male adipose-lineage ERα-mutant mice are lean, have improved glucose sensitivity and are resistant to weight gain on a high-fat diet. Further, they are hypermetabolic, hyperphagic and hyperthermic, all consistent with a brown phenotype. Together, these findings indicate that ERα cell autonomously regulates adipose lineage commitment, brown fat and smooth muscle cell formation, and systemic metabolism, in a manner relevant to prevalent metabolic diseases. Adipose tissues play diverse roles including serving as a central nexus of metabolic communication and control, an arbiter of thermoregulation, a buffer against trauma and the cold and a regulator of reproduction and satiety [1] , [2] . The key roles that adipose tissues play in metabolism are highlighted by the myriad complications, such as diabetes, hyperlipidemia, cancer and cardiovascular disease, associated with too much or too little fat [3] . In addition to roles as an energy repository, adipose tissues are an endocrine organ controlling appetite, glucose homeostasis, insulin sensitivity, fertility, ageing and even body temperature [4] , [5] . In mammals, adipose depots form in utero , in the peri-partum period, and are continually maintained throughout life [2] , [4] . Adipocytes are of two broad histological and functional types: white adipose tissues (WAT) that store energy, and brown adipose tissues (BATs) that dissipate energy and generate heat [5] . White adipose depots are themselves subdivided, based on gross anatomic location, into subcutaneous and visceral depots that contribute differently to metabolism [6] . A primary role of brown adipocytes, which express a molecular thermogenic programme, is likely in the neonatal period when thermoregulation is challenged, and it has been difficult to identify classical brown adipose in human adults, as well as in many other adult mammals [5] . Yet, brown adipocytes are also present in adult mammals, including mice and humans, but these appear to be of distinct lineage from those present in the neonatal period [5] , [6] , [7] . These adult thermogenic adipocytes, variously termed inducible BAT, beige or brite adipocytes, can be induced in adult white adipose depots by cold exposure, adrenergic agonists or irisin [8] , [9] , [10] . These new brown adipocytes have drawn increasing attention as their inherent energy dissipating properties have potential for weight loss [9] , [11] . Gonadal or ‘sex’ steroids, for example oestrogen or testosterone, are potent endogenous regulators of adiposity, adipose remodelling and metabolism [12] . For example, women tend to have more total and subcutaneous fat than men [13] . This oestrogen-dependent ‘female’ pattern of fat distribution is thought to be metabolically protective, as visceral fat, increased in males, is associated with poor metabolic outcomes [14] , [15] , [16] . The increased fat mass observed during female puberty may be secondary to an activated adipose stem cell compartment; oestrogen stimulates proliferation of cultured or primary preadipocytes [17] , [18] , [19] . After menopause, and the decline in circulating oestrogen, rodents and humans develop increased fat mass, glucose intolerance and abnormalities in temperature regulation; oestrogen replacement therapy blunts these effects [20] , [21] . Oestrogen actions are primarily mediated by oestrogen receptors (ERα, β), nuclear hormone receptors that act as ligand-dependent transcription factors [17] , [20] , [22] . A variety of genetic studies indicate that many of the effects of oestrogen on metabolism are mediated by the central nervous system (CNS) actions of ERα, although the liver, muscles and pancreas may contribute as well [20] , [23] . For example, whole-body, mature adipocyte, brain or hypothalamic ERα mutants have insulin resistance, impaired glucose tolerance and increased adiposity that may in part be secondary to reduced metabolic rate [23] , [24] , [25] . These mouse strains displayed many of the metabolic features triggered by menopause, although not all; many of the conditional brain mutants are reported to have decreased body temperature rather than the increases seen in oestrogen-deficient states [14] . Fat remodelling, such as that due to obesity and sex steroids, was primarily thought to be a hypertrophic phenomenon [26] . However, recent studies, including indications that the alterations of fat mass observed in high-fat diet (HFD) or in ERα mutants are secondary to increased adipocyte number, challenge this notion with hyperplasia and formation of new white adipocytes likely playing a greater role in adipose biology than previously considered [2] , [17] , [22] , [24] , [27] . These studies highlight roles of adipose progenitor cells as a source of white adipocytes, and some evidence indicates that these cells reside in the mural compartment of adipose depot blood vessels [28] , [29] . We developed a series of reagents, termed AdipoTrak, to visualize and manipulate gene expression of adipose progenitor cells in vivo , and to follow their descendants as they divide, migrate, differentiate or change fate [29] , [30] . AdipoTrak is an inducible marking and tracking system that combines a PPARγ tTA ‘knock-in’ allele with complementary reporters (for example, TRE-H2B-GFP, R26R) and advanced nucleotide labelling [29] , [30] , [31] , [32] . PPARγ has dosage-sensitive functions, including roles in metabolism; the AdipoTrak knock-in creates PPARγ heterozygosity, which has been shown to reduce adiposity and insulin resistance, with potential attendant consequences [33] . Studies show that AdipoTrak labels cells in the stromal vascular fraction (SVF), known to contain adipose progenitor cells, but not adipocytes, that self-renew, proliferate, enter quiescence and retain label, and that differentiate in vivo , in transplants and in vitro , the hallmarks of endogenous progenitor cells. AdipoTrak is expressed in adipose progenitor cells and also throughout adipose lineage specification into adipocytes. Thus, AdipoTrak allows delineation of many aspects of the adipose lineages, including the progenitor cell pool, adipocyte formation and adipose life cycle and turnover [29] , [34] . Of note, PPARγ is endogenously expressed in many cell and tissue types and is not specific for the adipose lineage. Further, some of these other cell types play key roles in metabolism. Therefore, as AdipoTrak is expressed in some of these other cell types as well, including those with metabolic actions, aspects of the adipose lineage or metabolic effects of AdipoTrak-driven mutations may be due to non-adipose lineage autonomous actions. However, various stromal vascular (SV) cells, fluorescence-activated cell sorting (FACS)-isolated progenitor and organotypic assays help address potential autonomy [35] , [36] , [37] , [38] . To attempt to elucidate a potential role of oestrogen signalling in the adipose progenitor cells and throughout adipose lineage specification, we generated AdipoTrak, ERα fl/fl conditional knockout mice (AT-ERαKO). Paradoxically and unlike whole-body or brain ERα mutants, AT-ERαKO mice displayed reduced adipogenic potential and fat mass, improved glucose sensitivity, resistance to HFD and increased metabolic rate and body temperature. The mutant cells rather appeared reprogrammed, differentiating into either a smooth muscle or a brown adipocyte lineage, a mechanism that involves, at least in part, activated transforming growth factor-β (TGFβ) signalling. Together, the data indicate that adipose progenitor cells have in vivo multi-lineage potential that is in part regulated by ERα, in a manner that may be effective for obesity, menopause and attendant metabolic dysfunction. Oestrogen regulates the adipose progenitor cell compartment Adipose progenitor cells are a minority component of the adipose SVF that also contains immune cells, fibroblasts, nerves, smooth muscle cells and endothelial cells, the latter two highlighting a potential perivascular adipose progenitor cell niche [29] . To determine whether oestrogen might regulate the adipose progenitor compartment, we performed sham operations or ovariectomy (OVX) on AdipoTrak mice in which the adipose progenitor compartment and lineage are marked with various reporters, for example a nuclear GFP or an indelible Rosa26-reporter [29] . Three weeks later, after oestrogen levels declined, we randomized control and OVX female to vehicle or BrdU, a synthetic nucleoside analogue that is incorporated into DNA during mitosis [30] . We then isolated stromal vascular cells and quantified, using flow cytometric methods, progenitor cell number (GFP + ) and progenitor cell proliferation (GFP + , BrdU + ) in this oestrogen-deficient setting; the mice that never received BrdU served as gating controls. We found that following OVX, a model of oestrogen deficiency, adipose progenitor cell proliferation and number were increased ( Fig. 1a ). 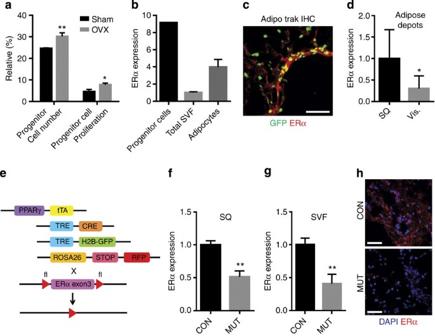Figure 1: ERα signalling and conditional deletion in adipose progenitor cells and throughout lineage specification. (a) AdipoTrak-GFP mice were randomized to sham or ovariectomy (OVX), 3 weeks later both groups were randomized to vehicle (gating controls) or BrdU, and then the number of progenitor cells and their BrdU incorporation was quantified with flow cytometry (n=5). (b) Real-time quantification of ERα mRNA expression in FACS-isolated progenitor cells, in total stromal vascular fraction (SVF) and in adipocytes (n≥10). (c) ERα immunohistochemistry of AdipoTrak-GFP adipose depot histological sections: progenitor cell nuclei are labelled green, ERα staining in red and co-expression in yellow. Scale bar, 100 μm. (d) Real-time analyses of ERα mRNA expression in subcutaneous (SQ) and visceral (Vis.) depots of female mice (n=6). (e) Schema of AdipoTrak progenitor and lineage deletion of ERα with lineage marking. In PPARγ-positive cells, tTA is translated and binds to a transgenic tet-response element (TRE), inducing Cre expression, ERα deletion, indelible R26R marking and lineage-sensitive nuclear GFP marking. Maroon arrowheads represent LoxP sites. (f,g) Real-time analyses of ERα mRNA expression in control and AT-ERαKO mutant subcutaneous white adipose tissue (SQ) (f) and in isolated SVF (g).n≥8/genotype. (h) ERα immunofluorescence of control and AT-ERαKO IWAT. Upper panel is section of control inguinal white adipose tissue (IWAT). Lower panel is section of AT-ERαKO IWAT. DAPI labels nuclei blue, ERα expression is in red. Scale bar, 100 μm. Error bars indicate s.e.m. Statistical significance assessed by two-tailed Student’st-test, *P<0.05, **P<0.01. Figure 1: ERα signalling and conditional deletion in adipose progenitor cells and throughout lineage specification. ( a ) AdipoTrak-GFP mice were randomized to sham or ovariectomy (OVX), 3 weeks later both groups were randomized to vehicle (gating controls) or BrdU, and then the number of progenitor cells and their BrdU incorporation was quantified with flow cytometry ( n =5). ( b ) Real-time quantification of ERα mRNA expression in FACS-isolated progenitor cells, in total stromal vascular fraction (SVF) and in adipocytes ( n ≥10). ( c ) ERα immunohistochemistry of AdipoTrak-GFP adipose depot histological sections: progenitor cell nuclei are labelled green, ERα staining in red and co-expression in yellow. Scale bar, 100 μm. ( d ) Real-time analyses of ERα mRNA expression in subcutaneous (SQ) and visceral (Vis.) depots of female mice ( n =6). ( e ) Schema of AdipoTrak progenitor and lineage deletion of ERα with lineage marking. In PPARγ-positive cells, tTA is translated and binds to a transgenic tet-response element (TRE), inducing Cre expression, ERα deletion, indelible R26R marking and lineage-sensitive nuclear GFP marking. Maroon arrowheads represent LoxP sites. ( f , g ) Real-time analyses of ERα mRNA expression in control and AT-ERαKO mutant subcutaneous white adipose tissue (SQ) ( f ) and in isolated SVF ( g ). n ≥8/genotype. ( h ) ERα immunofluorescence of control and AT-ERαKO IWAT. Upper panel is section of control inguinal white adipose tissue (IWAT). Lower panel is section of AT-ERαKO IWAT. DAPI labels nuclei blue, ERα expression is in red. Scale bar, 100 μm. Error bars indicate s.e.m. Statistical significance assessed by two-tailed Student’s t -test, * P <0.05, ** P <0.01. Full size image To investigate a possible role of ERα within adipose progenitors per se (for example, cell autonomous), we quantified ERα expression in flow-sorted AdipoTrak-marked (GFP + ) adipose progenitor cells, in the entire SVF compartment (GFP − and GFP + ) and in floated adipocytes. ERα was expressed in all three compartments with the lowest levels in the SVF, intermediate levels in adipocytes and the highest expression in the flow-purified progenitor compartment ( Fig. 1b ). Immunohistochemical (IHC) studies also show high ERα expression in adipose progenitor cells that reside in the perivascular niche ( Fig. 1c ). Furthermore, and consistent with the literature [39] , ERα expression was higher in subcutaneous WAT depots as compared with the visceral WAT depots ( Fig. 1d ). Adipose lineage ERα-mutant mice are lean To explore potential ERα cell autonomous functions in adipose progenitor cells and adipose lineage specification as suggested by the OVX and ERα expression studies ( Fig. 1a–d ), we combined AdipoTrak and an ERα conditional allele, generating AT-ERαKO mutants (PPARγ-tTA; TRE-Cre; ERα fl/fl , Fig. 1e ); alternative genotypes lacking either TRE-Cre or conditional alleles served as littermate controls (for example, PPARγ-tTA; ERα fl/fl , PPARγ-tTA; TRE-Cre; ERα +/fl , or PPARγ-tTA; TRE-Cre; ERα +/+ ). Quantitative PCR (qPCR) and IHC studies indicated that the AT-ERαKO strategy was effective; ERα expression was reduced in adipose progenitor cells, in the SVF and in whole depots ( Fig. 1f–h ). The residual ERα expression is likely due to the heterogeneous composition of the SVF; our studies indicate that ERα deletion is efficient and relatively complete in the progenitor cells and the lineage ( Fig. 1g,h ). We next examined cohorts of normal chow fed 4-month-old female control and AT-ERαKO littermates for adipose and metabolic phenotypes. In contrast to reported whole-body or brain ERα-mutant females, AT-ERαKO females displayed significant reductions in body fat content and fat mass, with lower water mass, and a trend towards lower body weight and a stable lean compartment ( Fig. 2a–c ). Further, the size and mass of subcutaneous and visceral fat depots were significantly decreased in the AT-ERαKO mutant females compared with controls, with a lesser decrease in the visceral fat depots ( Fig. 2d–g ); other organs (for example, the kidney, spleen, muscle and heart) were not affected ( Fig. 2h ). These differences may indicate a higher dependency on ERα in the subcutaneous fat consistent with the elevated ERα expression in those depots ( Fig. 1d ). In concert with the reduced fat mass, molecular markers of the adipose lineage were significantly reduced in the subcutaneous and visceral adipose tissues of mutants ( Fig. 2i,j ). Despite lower adiposity, the adipocytes that are present in vivo displayed a relatively normal adipogenic profile ( Fig. 2k ). Aromatase levels were also lower in the mutants, but they were detectable indicating that controls and mutants may be able to produce oestrogen locally due to expression of the Aromatase gene ( Supplementary Fig. 1 ). Notably, we also observed a similar phenotype in male AT-ERαKO mutants, except that there are minimal phenotypic differences between the subcutaneous and visceral depots in male AT-ERαKO mutants; both types of depots demonstrated a similar reduction in mass ( Fig. 3a–i ). 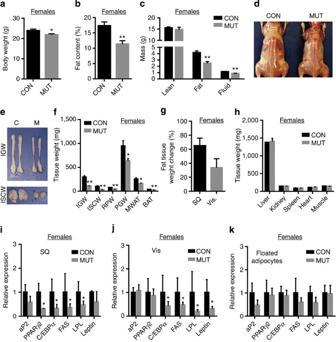Figure 2: AdipoTrak progenitor ERα-mutant female mice are lean. (a–c) Body weight (a), NMR body fat content (b) and lean, fat and fluid mass (c) of 4-month-old female control (CON) and AT-ERαKO (MUT) mice (n≥17 each) on normal chow diet. (d) Representative photograph of normal chow fed 4-month-old female control and AT-ERαKO littermates: adipose depots have whitish hue. (e) Representative photographs of inguinal (IGW) and interscapular (ISCW) white adipose tissue of 4-month-old female control (C) and AT-ERαKO siblings (M) fed normal chow. (f) Weight of indicated fat depots of 4-month-old female control and AT-ERαKO mutant siblings fed normal chow (n≥11). (g) Calculated percent reduction of fat tissue mass in female AT-ERαKO mutants compared with their controls: subcutaneous (SQ) depots (IGW+ISCW) and visceral (Vis.) depots (PGW+RPW). (h) Weight of indicated organs of chow fed control and AT-ERαKO female mice (n≥11). (i,j) Real-time analyses of adipose marker expression (aP2, PPARγ2, C/EBPα, FAS, LPL and Leptin) in control and AT-ERαKO subcutaneous (SQ,n=7 each) (i) and visceral (Vis.,n=7 each) (j) depots. (k) Floated adipocytes, isolated with density centrifugation, were analysed for expression of adipogenic markers (n≥4 each). Error bars indicate s.e.m. Statistical significance assessed by two-tailed Student’st-test, *P<0.05, **P<0.01. Figure 2: AdipoTrak progenitor ERα-mutant female mice are lean. ( a – c ) Body weight ( a ), NMR body fat content ( b ) and lean, fat and fluid mass ( c ) of 4-month-old female control (CON) and AT-ERαKO (MUT) mice ( n ≥17 each) on normal chow diet. ( d ) Representative photograph of normal chow fed 4-month-old female control and AT-ERαKO littermates: adipose depots have whitish hue. ( e ) Representative photographs of inguinal (IGW) and interscapular (ISCW) white adipose tissue of 4-month-old female control (C) and AT-ERαKO siblings (M) fed normal chow. ( f ) Weight of indicated fat depots of 4-month-old female control and AT-ERαKO mutant siblings fed normal chow ( n ≥11). ( g ) Calculated percent reduction of fat tissue mass in female AT-ERαKO mutants compared with their controls: subcutaneous (SQ) depots (IGW+ISCW) and visceral (Vis.) depots (PGW+RPW). ( h ) Weight of indicated organs of chow fed control and AT-ERαKO female mice ( n ≥11). ( i , j ) Real-time analyses of adipose marker expression (aP2, PPARγ2, C/EBPα, FAS, LPL and Leptin) in control and AT-ERαKO subcutaneous (SQ, n =7 each) ( i ) and visceral (Vis., n =7 each) ( j ) depots. ( k ) Floated adipocytes, isolated with density centrifugation, were analysed for expression of adipogenic markers ( n ≥4 each). Error bars indicate s.e.m. Statistical significance assessed by two-tailed Student’s t -test, * P <0.05, ** P <0.01. 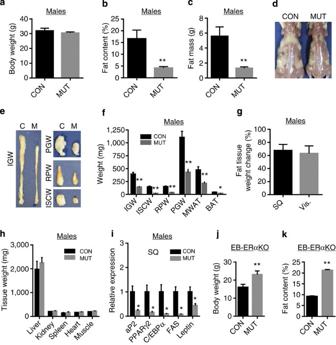Figure 3: AdipoTrak progenitor ERα mutant male mice are lean. (a–c) Body weight (a), NMR body fat content (b) and fat mass (c) of 4-month-old male control (CON) and AT-ERαKO (MUT) mice (n≥6 each) on normal chow diet. (d) Representative photograph of normal chow fed 4-month-old male control and AT-ERαKO littermates; adipose depots display whitish hue. (e) Representative photographs of inguinal (IGW), perigonadal (PGW), retroperitoneal (RPW) and interscapular (ISCW) white adipose tissue of 4-month-old male control (C) and AT-ERαKO siblings (M) fed normal chow. (f) Weight of indicated fat depots of 4-month-old male control and AT-ERαKO mutant siblings fed normal chow (n=5–9). (g) Calculated percent reduction of fat depot mass in AT-ERαKO male mutants compared with controls: subcutaneous (SQ) depots (IGW+ISCW) and visceral (Vis.) depots (PGW+RPW). (h) Weight of indicated organs of chow fed control and AT-ERαKO male mice (n=5–9). (i) Real-time analyses of adipose marker levels (aP2, PPARγ2, C/EBPα, FAS and Leptin) in control and AT-ERαKO IGW (n=5–13 each). (j,k) Body weight (j) and NMR fat content (k) of 4-month-old female control and epiblast-generated Sox2-Cre; ERαKO mice (EB-ERαKO,n≥10 each) fed normal chow. Error bars indicate s.e.m. Statistical significance assessed by two-tailed Student’st-test, *P<0.05, **P<0.01. Full size image Figure 3: AdipoTrak progenitor ERα mutant male mice are lean. ( a – c ) Body weight ( a ), NMR body fat content ( b ) and fat mass ( c ) of 4-month-old male control (CON) and AT-ERαKO (MUT) mice ( n ≥6 each) on normal chow diet. ( d ) Representative photograph of normal chow fed 4-month-old male control and AT-ERαKO littermates; adipose depots display whitish hue. ( e ) Representative photographs of inguinal (IGW), perigonadal (PGW), retroperitoneal (RPW) and interscapular (ISCW) white adipose tissue of 4-month-old male control (C) and AT-ERαKO siblings (M) fed normal chow. ( f ) Weight of indicated fat depots of 4-month-old male control and AT-ERαKO mutant siblings fed normal chow ( n =5–9). ( g ) Calculated percent reduction of fat depot mass in AT-ERαKO male mutants compared with controls: subcutaneous (SQ) depots (IGW+ISCW) and visceral (Vis.) depots (PGW+RPW). ( h ) Weight of indicated organs of chow fed control and AT-ERαKO male mice ( n =5–9). ( i ) Real-time analyses of adipose marker levels (aP2, PPARγ2, C/EBPα, FAS and Leptin) in control and AT-ERαKO IGW ( n =5–13 each). ( j , k ) Body weight ( j ) and NMR fat content ( k ) of 4-month-old female control and epiblast-generated Sox2-Cre; ERαKO mice (EB-ERαKO, n ≥10 each) fed normal chow. Error bars indicate s.e.m. Statistical significance assessed by two-tailed Student’s t -test, * P <0.05, ** P <0.01. Full size image We next explored the integrity of the ERα conditional allele to address the possibility that allelic issues underlie the surprising findings that progenitor cell ERα mutants were paradoxically lean, rather than obese, as observed in whole-body mutants or oestrogen-deficient settings. We evaluated the conditional allele by ingressing an epiblast Cre driver, Sox2-Cre, to generate ERα-null progeny (EB-ERαKO=Sox2-Cre; ERα fl/fl ; EB= E pi B last) [40] . These EB-ERαKO mutants lacked ERα expression, were obese and also had other features of conventional whole-body nulls ( Fig. 3j,k ), supporting allele integrity. Adipose lineage ERα-mutant mice resist HFD To assess the response(s) of AT-ERαKO-mutant mice to caloric excess, we provided 2-month-old cohorts of control and AT-ERαKO female littermates with 12 weeks of HFD. We weighed the mice weekly; controls and AT-ERαKO mutants had roughly equal rates of weight gain and slightly lower body weights at the end point ( Fig. 4a and Supplementary Fig. 2a ). However, nuclear magnetic resonance (NMR) fat content analyses showed significantly lower adiposity in the AT-ERαKO mutants, a trend towards higher lean mass, and the sizes of the fat depots were decreased compared with controls ( Fig. 4b,e ). Thus, HFD triggers an increase in AT-ERαKO mutant fat content and depot mass, yet overall adiposity is lower than controls on HFD ( Fig. 4b–d ). Other organs had normal weights ( Supplementary Fig. 2b ). The HFD fed AT-ERαKO mutants also exhibited a reduced adipogenic gene expression profile compared with controls ( Fig. 4f ). Together, these data indicate that AT-ERαKO-mutant mice have reduced fat mass and resist HFD-induced obesity. 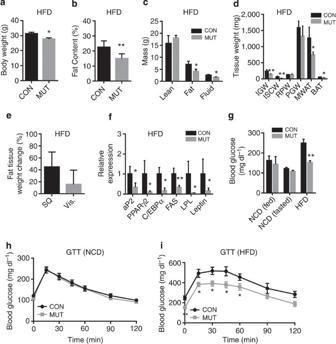Figure 4: AdipoTrak progenitor ERα-mutant mice resist high-fat diet and have improved glucose sensitivity. (a–c) Body weight (a), NMR body fat content (b) and lean, fat and fluid mass (c) of 4- to 5-month-old female control and AT-ERαKO mice (n=6 each) fed 10 weeks of high-fat diet (HFD). (d) Weights of indicated fat depots of 4- to 5-month-old female control and AT-ERαKO mutant siblings fed HFD (n≥6 each). (e) Calculated percent reduction of fat tissue weight in AT-ERαKO female mutants as compared with their controls under HFD setting: subcutaneous (SQ) depots (IGW+ISCW) and visceral (Vis.) depots (PGW+RPW). (f) Real-time analyses of adipose marker mRNA (aP2, PPARγ2, C/EBPα, FAS, LPL and Leptin) in control and AT-ERαKO IGW under HFD setting (n≥6 each). (g) Blood glucose levels of control and AT-ERαKO female littermates on normal chow diet (NCD, fed or fasted) or HFD (fasted) (n≥6 each). (h,i) Glucose tolerance tests (GTTs) of NCD (h) and HFD fed (i) 4- to 5-month-old control and AT-ERαKO mutant female siblings (n≥10/genotype). Error bars indicate s.e.m. Statistical significance assessed by two-tailed Student’st-test, *P<0.05, **P<0.01. Figure 4: AdipoTrak progenitor ERα-mutant mice resist high-fat diet and have improved glucose sensitivity. ( a – c ) Body weight ( a ), NMR body fat content ( b ) and lean, fat and fluid mass ( c ) of 4- to 5-month-old female control and AT-ERαKO mice ( n =6 each) fed 10 weeks of high-fat diet (HFD). ( d ) Weights of indicated fat depots of 4- to 5-month-old female control and AT-ERαKO mutant siblings fed HFD ( n ≥6 each). ( e ) Calculated percent reduction of fat tissue weight in AT-ERαKO female mutants as compared with their controls under HFD setting: subcutaneous (SQ) depots (IGW+ISCW) and visceral (Vis.) depots (PGW+RPW). ( f ) Real-time analyses of adipose marker mRNA (aP2, PPARγ2, C/EBPα, FAS, LPL and Leptin) in control and AT-ERαKO IGW under HFD setting ( n ≥6 each). ( g ) Blood glucose levels of control and AT-ERαKO female littermates on normal chow diet (NCD, fed or fasted) or HFD (fasted) ( n ≥6 each). ( h , i ) Glucose tolerance tests (GTTs) of NCD ( h ) and HFD fed ( i ) 4- to 5-month-old control and AT-ERαKO mutant female siblings ( n ≥10/genotype). Error bars indicate s.e.m. Statistical significance assessed by two-tailed Student’s t -test, * P <0.05, ** P <0.01. Full size image AT-ERαKO mutants show improved systemic glucose sensitivity Oestrogen signalling regulates glucose homeostasis; whole-body and brain mutant animals as well as post-menopausal women show relative glucose insensitivity [20] , [23] , [24] . To probe potential physiological consequences of the AT-ERαKO mutation, we monitored blood glucose concentration in the fasted and fed state in control and AT-ERαKO female littermates. In either setting, control and mutant sera glucose concentrations were approximately the same ( Fig. 4g ). Yet the AT-ERαKO mutation blunted HFD-induced hyperglycemia ( Fig. 4g ). We further dissected glucose homeostasis through dynamic testing of adult control and mutant female cohorts fed a normal or a HFD. On normal chow, the mutants displayed normal glucose and insulin sensitivity and basal levels of insulin ( Fig. 4h , Supplementary Fig. 2c,d ). However, HFD fed AT-ERαKO female mutants had significantly improved glucose tolerance ( Fig. 4i ). Although insulin tolerance had a non-significant trend towards improvement ( Supplementary Fig. 2e ), other yet undiscovered factors might account for the improved glucose sensitivity under HFD ( Fig. 4i , Supplementary Fig. 2c ). AT-ERαKO mutants have an altered progenitor compartment To attempt to unravel a possible progenitor cell-autonomous effect(s) of the AT-ERα mutation, we ingressed into the AT-ERαKO mice, a TRE-H2B-GFP reporter (AT-ERαKO-GFP=PPARγ-tTA; TRE-Cre; ERα fl/fl ; TRE-H2B-GFP) that expresses a fate-sensitive nuclear GFP; expression is abrogated by a lineage change [29] . To evaluate whether the ERα mutation might alter the number of adipose progenitor cells, we explanted control and mutant subcutaneous adipose depots (high ERα expression, expressive phenotype) and examined them with fluorescent microscopy. We found that the mutants had a marked diminution in GFP expression ( Fig. 5a ), supporting the notion that loss of ERα alters progenitor cell function, which may account for the adipocyte phenotype (for example, altered adipocyte number, life cycle, gene expression, and so on.) that we observed in the mutant mice ( Figs 2 , 3 , 4 ). To explore this possibility in greater detail, we quantified progenitor cell number with flow cytometry. The flow profiles indicated a significant reduction in the AT-ERαKO-GFP mutant adipose progenitor pool ( Fig. 5b,c ). HFD appears to be able to compensate for this effect, indicating that the progenitor cell pool remains responsive to stimuli ( Supplementary Fig. 2f ). 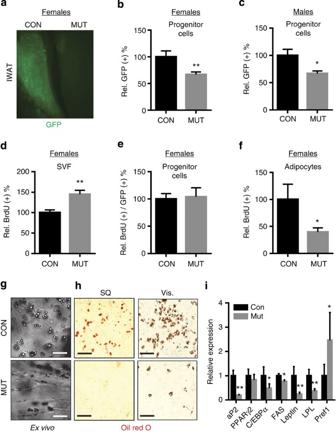Figure 5: AT-ERαKO mutants have an altered progenitor compartment, reduced progenitor cell number and inhibited adipogenic potential. (a) GFP-fluorescent images of inguinal adipose depots of 4-month-old female control and AT-ERαKO-GFP littermates. (b,c) SV cells were isolated from adipose depots of 4-month-old control and AT-ERαKO-GFP female (b) and male (c) littermates on normal chow. The SV cells were subjected to flow cytometry to quantify progenitor cell number (relative GFP %). The GFP+gates were based on controls with the TRE-H2B-GFP reporter alone (n≥6/genotype). (d,e) Four-month-old female control and AT-ERαKO-GFP littermates were provided BrdU, and then BrdU incorporation into total SV cells (d) and GFP+ progenitor cells (e) was quantified with flow cytometry (n≥4/genotype). (f) Four-month-old female control and AT-ERαKO littermates were provided BrdU for 3 weeks, and then BrdU incorporation into floated adipocytes, as an indicator of adipogenic differentiation, was quantified with flow cytometry (n≥5/genotype). (g) Control and AT-ERαKO IGW adipose depots were explanted, placed into organotypic culture and 1 week later photographed under pseudo-Nomarki microscopy to assess adipogenic potential. Controls show birefringent adipocytes, mutants show tubular networks, but not adipocytes. Scale bar, 100 μm. (h,i) SV cells of control and AT-ERαKO subcutaneous (SQ) and visceral (Vis.) depots were isolated, cultured and adipogenically induced. Adipogenesis was assayed with Oil Red O. (h, fat stains red, scale bar=100 μm) and qPCR (i) of adipogenic and adipocyte (PPARg, C/EBPa, aP2, Leptin, FAS and LPL) as well as preadipocyte (Pref-1) markers (n≥5/genotype). Error bars indicate s.e.m. Statistical significance assessed by two-tailed Student’st-test, *P<0.05, **P<0.01. Figure 5: AT-ERαKO mutants have an altered progenitor compartment, reduced progenitor cell number and inhibited adipogenic potential. ( a ) GFP-fluorescent images of inguinal adipose depots of 4-month-old female control and AT-ERαKO-GFP littermates. ( b , c ) SV cells were isolated from adipose depots of 4-month-old control and AT-ERαKO-GFP female ( b ) and male ( c ) littermates on normal chow. The SV cells were subjected to flow cytometry to quantify progenitor cell number (relative GFP %). The GFP + gates were based on controls with the TRE-H2B-GFP reporter alone ( n ≥6/genotype). ( d , e ) Four-month-old female control and AT-ERαKO-GFP littermates were provided BrdU, and then BrdU incorporation into total SV cells ( d ) and GFP+ progenitor cells ( e ) was quantified with flow cytometry ( n ≥4/genotype). ( f ) Four-month-old female control and AT-ERαKO littermates were provided BrdU for 3 weeks, and then BrdU incorporation into floated adipocytes, as an indicator of adipogenic differentiation, was quantified with flow cytometry ( n ≥5/genotype). ( g ) Control and AT-ERαKO IGW adipose depots were explanted, placed into organotypic culture and 1 week later photographed under pseudo-Nomarki microscopy to assess adipogenic potential. Controls show birefringent adipocytes, mutants show tubular networks, but not adipocytes. Scale bar, 100 μm. ( h , i ) SV cells of control and AT-ERαKO subcutaneous (SQ) and visceral (Vis.) depots were isolated, cultured and adipogenically induced. Adipogenesis was assayed with Oil Red O. ( h , fat stains red, scale bar=100 μm) and qPCR ( i ) of adipogenic and adipocyte (PPARg, C/EBPa, aP2, Leptin, FAS and LPL) as well as preadipocyte (Pref-1) markers ( n ≥5/genotype). Error bars indicate s.e.m. Statistical significance assessed by two-tailed Student’s t -test, * P <0.05, ** P <0.01. Full size image The diminished AT-ERαKO adipose progenitor cell pool under normal diet might be due to reduced progenitor cell proliferation. Adipose progenitor cells appear to constitute a subset of the mural compartment (for example, pericytes, vascular smooth muscle cells) [29] , and various reports indicate that depending on context oestrogen inhibits vascular smooth muscle proliferation [41] , [42] , [43] , [44] , [45] . Loss of ERα signalling, therefore, might be predicted to increase progenitor (mural cell) proliferation; yet we observed a reduction in adipose progenitor cell number in the mutants. To test proliferative rates, we provided BrdU. Three weeks later, we explanted subcutaneous adipose depots and isolated total SVF, progenitor cells, as well as floated adipocytes. We found that mutant, compared with control, SVF incorporated more BrdU, indicating increased proliferation of the mutant SV compartment ( Fig. 5d ). To determine whether the progenitor compartment per se was also hyperproliferative, we again measured levels of BrdU, but specifically within the progenitor compartment by quantifying BrdU + , GFP + double-positive cells. We found that proliferation was roughly equal in mutants and controls ( Fig. 5e ). We also examined progenitor cell apoptosis, but Annexin V flow profiles were unchanged in the mutants (not shown) [30] . Together the data indicated that the number of adipose progenitor cells is reduced, but this reduction does not appear secondary to altered progenitor cell proliferation or progenitor cell death. We next began to evaluate the degree or rate of adipocyte formation as a possible contributor to the reduced progenitor cell quantity. To that end, we repeated the BrdU protocols, but after 3 weeks we isolated floated adipocytes with density centrifugation and examined their BrdU incorporation as an indicator of adipogenic differentiation, as described in ref. 30 . We found that in vivo adipocyte formation was significantly reduced by the ERα mutation ( Fig. 5f ). Although the blockade in white adipogenesis does not explain the reduced progenitor cell number, it might account for the reduced adiposity observed in the AT-ERαKO mice. To further assess possible changes in adipocyte differentiation in the mutants, we placed control and AT-ERαKO adipose depot explants into organotypic culture [46] and incubated the explants in media containing insulin, a hormone that stimulates adipocyte formation. After 1 week, we examined the explants with pseudo-Nomarski microscopy. Cells from control explants contained multiple-lipid laden cells, indicating robust adipogenic differentiation ( Fig. 5g ). In contrast, the mutant explants did not form adipocytes and instead differentiated into a network of capillary-like structures ( Fig. 5g ). To examine whether the apparent reduction in adipogenic potential was due to an altered microenvironment or a cell autonomous (for example, progenitor cell specific) effect, we isolated control and AT-ERαKO SV cells, and incubated them in adipogenic induction media. On the basis of bright field microscopy, Oil Red O stains and qPCR analyses, adipogenic differentiation was blunted in AT-ERαKO mutants ( Fig. 5h,i ). For example, expression of adipogenic transcription factors and adipokines were low, while levels of Pref-1, an adipogenic inhibitor [47] , were high, in cultured mutant cells, supporting a differentiation block ( Fig. 5i ). Together, the data indicate that the AT-ERαKO adipose progenitor compartment is altered, the progenitor cell number is reduced and the evolution of progenitor cells into white adipocytes is inhibited. AT-ERαKO adipose depots have an angiogenic phenotype To attempt to dissect the cellular basis of the reduced adiposity phenotypes, we histologically analysed subcutaneous, visceral and brown adipose depots of control and AT-ERαKO female and male siblings fed normal chow. Haematoxylin and eosin-stained sections showed that the mutants had distorted micro-architecture ( Fig. 6a,b ). A prominent feature was a marked increase in blood vessel-like structures in mutant subcutaneous adipose tissues that resonated with the organotypic data, indicating exuberant tubulogenesis of isolated AT-ERαKO explants ( Figs 5g and 6a,b ). This altered micro-architecture was also observed under HFD and interestingly in whole-body EB-ERαKO in spite of their high adiposity ( Fig. 6c,d ), supporting the generality of the effect. Many blood vessels in the AT-ERαKO mutants had an abnormal appearance, with increases in the vascular smooth muscle compartment that in some cases was quite marked ( Fig. 6a–c ). However, vessels in other tissues did not appear to have a thickened vascular smooth muscle compartment, and we did not detect vascular leak ( Supplementary Fig. 3a,b ). Notably, IHC analyses (smooth muscle, SMA; endothelium, PECAM) also showed a significant increase in the vasculature in AT-ERαKO depots compared with controls ( Fig. 6e ). Further, the SMA stains support the notion that some mutant vessels have an exaggerated vascular smooth muscle compartment ( Fig. 6e ). The observed angiogenic phenotype was also supported by flow cytometry and qPCR studies that show increased expression of vascular markers (for example, SMA, PECAM) and angiogenic factors (for example, VEGF, Ang, FGF-2, and so on), which are often expressed by activated mural cells to drive endothelial proliferation ( Fig. 6f,g , Supplementary Fig. 3c ) [48] , [49] . 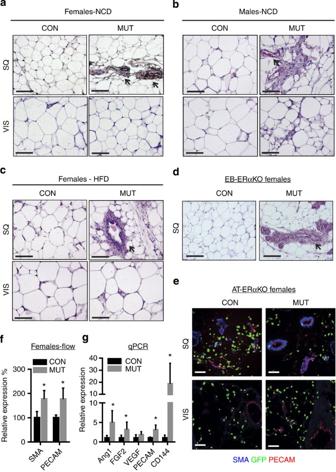Figure 6: AT-ERαKO mutants show enhanced angiogenic phenotype. (a–c) Haematoxylin and eosin (H&E)-stained histological sections of representative subcutaneous (SQ) and visceral (VIS) WAT 4-month-old control and AT-ERαKO mice. Females (a) and males (b) on normal chow diet (NCD) or females after 10 weeks of high fat-diet (HFD) (c). Black arrows indicate extensive vascular morphology. Scale bar=100 μm. (d) H&E-stained histological sections of representative subcutaneous WAT of female control and EB-ERαKO mice fed normal chow. Arrow indicates an abnormal blood vessel. Scale bar=100 μm. (e) Immunofluorescent analyses of SQ and VIS adipose tissue sections of 4-month-old female control and AT-ERαKO mutants stained for GFP (green, adipose lineage), PECAM (red, endothelium) and SMA (blue, mural). Scale bar=50 μm. (f) The levels of SMA and PECAM in the SVF of a 4-month-old female control and AT-ERαKO were flow cytometrically quantified and plotted (n≥4). (g) The mRNA levels of various vascular/angiogenic markers expressed in the SVF of 4-month-old female control and AT-ERαKO littermates were quantified with qPCR (n≥5). Error bars indicate s.e.m. Statistical significance assessed by two-tailed Student’st-test, *P<0.05. Figure 6: AT-ERαKO mutants show enhanced angiogenic phenotype. ( a – c ) Haematoxylin and eosin (H&E)-stained histological sections of representative subcutaneous (SQ) and visceral (VIS) WAT 4-month-old control and AT-ERαKO mice. Females ( a ) and males ( b ) on normal chow diet (NCD) or females after 10 weeks of high fat-diet (HFD) ( c ). Black arrows indicate extensive vascular morphology. Scale bar=100 μm. ( d ) H&E-stained histological sections of representative subcutaneous WAT of female control and EB-ERαKO mice fed normal chow. Arrow indicates an abnormal blood vessel. Scale bar=100 μm. ( e ) Immunofluorescent analyses of SQ and VIS adipose tissue sections of 4-month-old female control and AT-ERαKO mutants stained for GFP (green, adipose lineage), PECAM (red, endothelium) and SMA (blue, mural). Scale bar=50 μm. ( f ) The levels of SMA and PECAM in the SVF of a 4-month-old female control and AT-ERαKO were flow cytometrically quantified and plotted ( n ≥4). ( g ) The mRNA levels of various vascular/angiogenic markers expressed in the SVF of 4-month-old female control and AT-ERαKO littermates were quantified with qPCR ( n ≥5). Error bars indicate s.e.m. Statistical significance assessed by two-tailed Student’s t -test, * P <0.05. Full size image The adipose lineage ERα deletion induces a fate change The reduced adipose progenitor cell number in the face of inhibited adipogenic differentiation, normal progenitor cell proliferation and apoptosis could be accounted for, if AT-ERαKO cells were reprogrammed to differentiate into an alternative fate(s). To assess a possible lineage transformation, for example into the expanded mural compartment observed in histological sections, we examined the potential of control and AT-ERαKO adipose depot explants to generate smooth muscle cells in an organotypic setting. We cultured explants of control and mutant adipose depots for 1 week (as in Fig. 5g ) and then extended the culture duration for a second week, during which we included insulin in the media in attempt to trigger differentiation. After the 2 weeks in culture, we examined newly generated cells that emanated from the explant for morphology and SMA expression. We found that descendants of control depots generated adipocytes, but mutant progeny did not ( Fig. 7a ), consistent with the differentiation blockade described above ( Fig. 5g–i ). Rather, mutant cells generated a tubular, vessel-like network ( Fig. 7a ), in which innumerable cells displayed mural cell morphology, and, consistent with that, the cells derived from mutant, but not control, depots expressed smooth muscle actin in a prototypic fibre arrangement ( Fig. 7b ). To explore the possibility that this was a cell autonomous (for example, progenitor specific) effect, we isolated AdipoTrak-GFP+ SV progenitor cells from control and AT-ERαKO depots, cultured them for 1 week and then examined GFP expression, adipogenesis and smooth muscle differentiation. Similar to the organotypic setting, isolated and cultured control progenitor cells underwent adipogenic differentiation, but the mutants did not ( Fig. 7c ). Rather, we found that mutant, but not control, progenitors appeared to be reprogrammed, differentiating into a smooth muscle lineage, illustrated by morphology and SMA immunostaining ( Fig. 7c,d ). Further, during the culture period, GFP expression was reduced compared with controls, indicating a lineage transformation ( Fig. 7d ). Together, these findings are consistent with a fate change as GFP reporter expression is adipose lineage specific [29] . To extend that notion, we examined cultured cells for expression of a panel of canonical mural cell markers, for example expression restricted isoforms of myosins or myosin kinases. We found that a battery of such smooth muscle/mural cell-associated markers had higher expression levels in the cultured mutant progenitor cells ( Fig. 7e ). To test the possibility that the increased smooth muscle phenotype observed in vivo might in part be due to an increased proliferation of these induced smooth muscle progenitors, we administered BrdU to 3-month-old control and AT-ERαKO siblings for 1 week, isolated the SVF and then analysed BrdU incorporation into the smooth muscle compartment. Flow cytometric analyses showed that the ERα-mutant depots had significantly increased smooth muscle proliferation ( Fig. 7f ). These studies indicate that ERα-deficient cells have a diminished capacity to function as white adipose progenitors, accounting for the reduction in GFP signal, and rather have changed fate and now function as smooth muscle lineage progenitors. 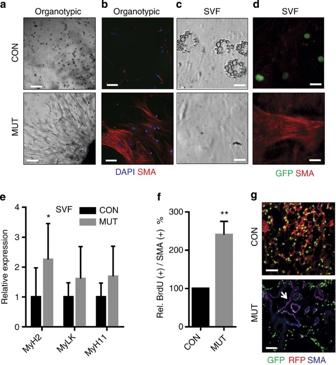Figure 7: The progenitor deletion of ERα induces a smooth muscle fate change. (a,b) Inguinal adipose depot explants of 4-month-old female control and AT-ERαKO mutants were organotypically cultured; after 1 week their lineage potential was assessed. (a) Control depots generated adipocytes with characteristic morphology, while AT-ERαKO depots developed vascular projections (sprouts). Scale bar=250 μm. (b) Smooth muscle lineage reprogramming was assessed with smooth muscle actin (SMA) immunofluorescence. DAPI (blue), SMA (red). Scale bar=100 μm. (c,d) Isolated SV cells, from 4-month-old female control and AT-ERαKO-GFP littermate depots, were cultured to confluence, and adipogenesis induced and assessed microscopically, scale bar=50 μm (c). Lineage reprogramming was assayed by GFP, a fate sensitive marker with expression extinguished by a fate change, and SMA immunofluorescence, scale bar=50 μm (d). (e) qPCR analyses of vascular smooth muscle markers (MyH2, MyH11 and MyLK) in cultured SVF obtained from inguinal WAT of control and AT-ERαKO female mice (n≥5). (f) Four-month-old female control and AT-ERαKO-GFP littermates were provided BrdU for 3 weeks, and proliferation of SMA-positive cells was examined with flow cytometric quantification (SMA+, BrdU+) (n=5). (g) Inguinal adipose tissues from 4-month-old AT-ERαKO-GFP-R26R-RFP double reporter mice (Control=PPARγ-tTA; TRE-Cre; ERα+/fl; TRE-H2B-GFP; R26R-tdTomato or Mutant=PPARγ-tTA; TRE-Cre; ERαfl/fl; TRE-H2B-GFP; R26R-tdTomato) were sectioned and stained for GFP (adipose lineage sensitive marker), RFP (lineage indelible marker) and SMA (mural cell marker). White arrow indicates SMA-expressing cells that derived from the AT-ERαKO-GFP adipose progenitors (RFP+) but that were reprogrammed and no longer express adipose lineage markers (GFP negative). Scale bar=100 μm. Error bars indicate s.e.m. or s.d. forFig. 7e. Statistical significance assessed by two-tailed Student’sttest, *P<0.05. **P<0.01. Figure 7: The progenitor deletion of ERα induces a smooth muscle fate change. ( a , b ) Inguinal adipose depot explants of 4-month-old female control and AT-ERαKO mutants were organotypically cultured; after 1 week their lineage potential was assessed. ( a ) Control depots generated adipocytes with characteristic morphology, while AT-ERαKO depots developed vascular projections (sprouts). Scale bar=250 μm. ( b ) Smooth muscle lineage reprogramming was assessed with smooth muscle actin (SMA) immunofluorescence. DAPI (blue), SMA (red). Scale bar=100 μm. ( c , d ) Isolated SV cells, from 4-month-old female control and AT-ERαKO-GFP littermate depots, were cultured to confluence, and adipogenesis induced and assessed microscopically, scale bar=50 μm ( c ). Lineage reprogramming was assayed by GFP, a fate sensitive marker with expression extinguished by a fate change, and SMA immunofluorescence, scale bar=50 μm ( d ). ( e ) qPCR analyses of vascular smooth muscle markers (MyH2, MyH11 and MyLK) in cultured SVF obtained from inguinal WAT of control and AT-ERαKO female mice ( n ≥5). ( f ) Four-month-old female control and AT-ERαKO-GFP littermates were provided BrdU for 3 weeks, and proliferation of SMA-positive cells was examined with flow cytometric quantification (SMA+, BrdU+) ( n =5). ( g ) Inguinal adipose tissues from 4-month-old AT-ERαKO-GFP-R26R-RFP double reporter mice (Control=PPARγ-tTA; TRE-Cre; ERα +/fl ; TRE-H2B-GFP; R26R-tdTomato or Mutant=PPARγ-tTA; TRE-Cre; ERα fl/fl ; TRE-H2B-GFP; R26R-tdTomato) were sectioned and stained for GFP (adipose lineage sensitive marker), RFP (lineage indelible marker) and SMA (mural cell marker). White arrow indicates SMA-expressing cells that derived from the AT-ERαKO-GFP adipose progenitors (RFP+) but that were reprogrammed and no longer express adipose lineage markers (GFP negative). Scale bar=100 μm. Error bars indicate s.e.m. or s.d. for Fig. 7e . Statistical significance assessed by two-tailed Student’s t test, * P <0.05. ** P <0.01. Full size image To further explore the notion that the AT-ERαKO mutant adipose lineage has changed fate and acquired the capacity to specify smooth muscle fates, we returned to the in vivo setting and introduced a conditional RFP reporter (R26R-tdTomato) into the AT-ERαKO-GFP-mutant background. Once activated in the adipose progenitors by AdipoTrak, the R26R-RFP allele indelibly marks adipose progenitor cells and all descendants with RFP whether they differentiate into the adipose lineage or they change fate and form a different lineage [49] , [50] . This is in contrast to the GFP reporter that is sensitive to lineage, and its expression is extinguished if the cells change fate and enter into a non-adipose lineage [34] . Integrating the two systems allows fate delineation; adipose lineages are indicated by RFP + , GFP + double positivity, while a lineage transformation produces RFP + , GFP − cells. Hence, we examined histological sections of AT-ERαKO-GFP-R26R-RFP double reporter mice (PPARγ-tTA; TRE-Cre; ERα fl/fl ; TRE-H2B-GFP; R26R-tdTomato) for expression of the reporters as well as markers of various other lineages for example, endothelial, PECAM; mural, SMA). We found that many SMA cells co-expressed the indelible RFP reporter, indicating they derived from the adipose progenitor compartment; yet, the GFP signal did not track with these double positive (RFP + , SMA + , GFP − ) cells ( Fig. 7g ). These data support the hypothesis that ERα, acting cell autonomously within adipose progenitor cells per se , plays an important role in adipose progenitor cell identity and function, and in its absence adipose progenitor cells appear to differentiate into an alternate fate(s), such as the vascular smooth muscle lineage. Lineage reprogramming is mediated by TGFβ signalling Various reports show that ERα activity often inhibits smooth muscle differentiation [41] , [42] , [43] , an effect that is consistent with the increase in smooth muscle formation that we observed in the adipose depots of AT-ERα mutants. Mechanistic studies link the oestrogen-dependent smooth muscle differentiation block to a downstream inhibition of TGFβ signalling, the latter promotes smooth muscle formation [50] , [51] , [52] . Consistent with the possibility that enhanced TGFβ signalling might be involved in the increased vascular smooth muscle differentiation observed in the AT-ERαKO mutants, AT-ERαKO adipose depots, which contain a wide array of cell types, expressed modestly, but significantly, increased levels of TGFβ ( Fig. 8a ). This heightened TGFβ expression appears to be transduced through the signalling cascade, as depots show (1) significantly altered expression of two direct TGFβ/SMAD4 target genes—ID1 and ATF3—that inhibit or promote fibrosis, respectively ( Fig. 8b ) [53] , and (2) increased Jun N-terminal kinase (JNK) phosphorylation ( Fig. 8c ) using adipose depot immunohistochemistry. Further, this effect appears to be restricted: cells in which we observed JNK phosphorylation were GFP + (in the adipose lineage), and we found a further enhancement (~3X) of TGFβ expression in cultured SV cells from AT-ERαKO mutants ( Fig. 8d ). 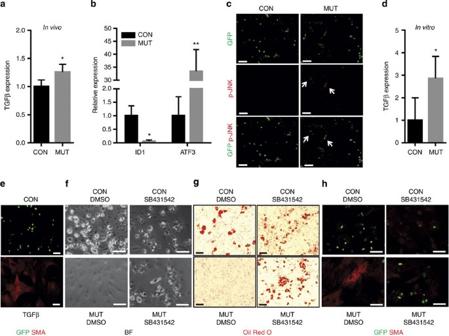Figure 8: An ERα—TGFβ switch regulates adipose potency. (a) TGFβ expression in mRNA extracted from adipose depots of 4-month-old female control and AT-ERαKO mutant siblings quantified with qPCR (n=5). (b) qPCR analyses of inguinal WAT TGFβ/SMAD4 target genes: ID1, transcription repressed by signalling, ATF3 transcription activated by TGFβ signalling (n≥7). (c) Phospho-JNK, TGFb target, immunohistochemistry of inguinal WAT of control and mutant AT-ERα mice. Arrow indicates co-localization of phospho-JNK and GFP+cells. Scale bar=50 μm. (d) TGFβ mRNA qPCR levels in cultured SV cells from 4-month-old female control and AT-ERαKO-mutant mice (n=5). (e) Differentiation of cultured control AdipoTrak-GFP SV cells in the presence or absence of 10 ng ml−1TGFβ. GFP marks adipocytes, red marks SMA+ smooth muscle cells. Scale bar=50 μm. (f–h) SV cells were isolated from 4-month-old female control and AT-ERαKO-GFP mutant siblings, were cultured, randomized to adipogenic induction medium containing either vehicle or a TGFβ inhibitor (SB431542, 10 μM), and adipogenic potential was assessed microscopically (f) or with Oil Red O staining (g). Scale bar=100 μm. Smooth muscle lineage reprogramming was assessed with SMA immunofluorescence and GFP expression (h); the latter is extinguished by a fate change. Scale bar=100 μm. Error bars indicate s.e.m. or s.d. forFig. 8d. Statistical significance assessed by two-tailed Student’st-test, *P<0.05, **P<0.01. Figure 8: An ERα—TGFβ switch regulates adipose potency. ( a ) TGFβ expression in mRNA extracted from adipose depots of 4-month-old female control and AT-ERαKO mutant siblings quantified with qPCR ( n =5). ( b ) qPCR analyses of inguinal WAT TGFβ/SMAD4 target genes: ID1, transcription repressed by signalling, ATF3 transcription activated by TGFβ signalling ( n ≥7). ( c ) Phospho-JNK, TGFb target, immunohistochemistry of inguinal WAT of control and mutant AT-ERα mice. Arrow indicates co-localization of phospho-JNK and GFP + cells. Scale bar=50 μm. ( d ) TGFβ mRNA qPCR levels in cultured SV cells from 4-month-old female control and AT-ERαKO-mutant mice ( n =5). ( e ) Differentiation of cultured control AdipoTrak-GFP SV cells in the presence or absence of 10 ng ml −1 TGFβ. GFP marks adipocytes, red marks SMA+ smooth muscle cells. Scale bar=50 μm. ( f – h ) SV cells were isolated from 4-month-old female control and AT-ERαKO-GFP mutant siblings, were cultured, randomized to adipogenic induction medium containing either vehicle or a TGFβ inhibitor (SB431542, 10 μM), and adipogenic potential was assessed microscopically ( f ) or with Oil Red O staining ( g ). Scale bar=100 μm. Smooth muscle lineage reprogramming was assessed with SMA immunofluorescence and GFP expression ( h ); the latter is extinguished by a fate change. Scale bar=100 μm. Error bars indicate s.e.m. or s.d. for Fig. 8d . Statistical significance assessed by two-tailed Student’s t -test, * P <0.05, ** P <0.01. Full size image To attempt to assess the possibility that the increased TGFβ expression and activated TGFβ signalling were functionally relevant to the observed smooth muscle fate change, we cultured AdipoTrak-GFP SVF (AT-GFP=PPARγ-tTA; TRE-H2B-GFP) in vehicle or TGFβ1 protein (10 ng ml −1 ) and then evaluated adipose (GFP + , green) and smooth muscle (SMA + , red) lineage formation. In this sufficiency test, we found that vehicle-treated samples contained numerous GFP + cells with adipose progenitor morphology and also bountiful adipocyte formation ( Fig. 8e ). In contrast, GFP expression and adipocyte formation were extinguished by TGFβ1 ligand, and the cells rather formed SMA + cells with a mural morphology ( Fig. 8e ), mirroring the effects observed in the AT-ERαKO-mutant SVF ( Fig. 7 ). We next turned to necessity tests to determine whether TGFβ signalling was required for the fate change observed in the AT-ERαKO mutants. We randomized control or AT-ERαKO mutant adipose SVF to culture in vehicle or in SB431542 (10 μM), a widely used TGFβ signalling inhibitor that is reported to have TGFβ-selective effects [54] . In vehicle, control progenitors differentiated into adipocytes (Birefringence in Fig. 8f , Oil Red O positive in Fig. 8g ), while the mutants did not; instead, they differentiated into SMA-expressing smooth muscle cells ( Fig. 8h ). Notably, the TGFβ inhibitor, which had no effect on control differentiation, reversed the ability of the mutant cells to form smooth muscle, and now the cells reacquired adipogenic potential and GFP expression ( Fig. 8h ). These data support the notion that ERα confers adipose progenitor cell identity in part by inhibiting TGF signalling; ERα loss activates TGFβ expression and signal transduction, which reprogrammes progenitor cells into alternative fates, such as the smooth muscle lineage. AT-ERα deletion reprogrammes progenitors into a brown lineage AT-ERαKO adipose depots, in addition to increased vasculature described above, demonstrated a chimeric or heterogeneous appearance with prominent clusters of multilocular cells in subcutaneous and less frequently in visceral depots that were not present in controls ( Fig. 9a,b ). Such multilocular cells can indicate formation of brown adipocytes, variously termed Brite, Beige or induced brown adipocytes, within WAT [9] . To unravel the possibility that AT-ERα deficiency might provoke a white to brown lineage transformation, we examine expression of relevant markers in control and AT-ERαKO interscapular classical brown and various white adipose depots [9] , [55] . qPCR analyses indicate that classical BAT and inguinal WAT from the AT-ERαKO-mutant female and male mice had significantly increased expression of a panel of genes associated with brown adipocytes including brown adipogenic factors (for example, PRDM16, PGC1α) as well as brown fat and thermogenic markers (for example, Cidea, EVA1, UCP1) ( Fig. 9c–e ). Further, both mutant inguinal WAT and BAT displayed increased UCP1 immunoreactivity ( Fig. 9f–h ). Co-localization of GFP + and UCP1 expression has been noted. These results support the notion that adipose lineage ERα signalling induces white adipose lineage commitment and that the lack of ERα alters the differentiation programme and the reprogrammed mutant cells now enter into the brown adipose lineage. 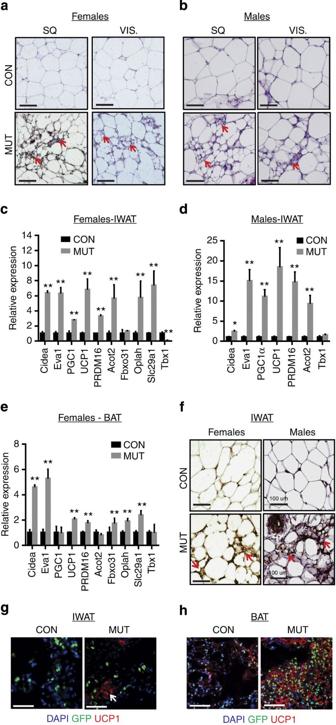Figure 9: Progenitor deletion of ERα: brown adipose reprogramming. (a,b) H & E-stained histological sections of subcutaneous (SQ) and visceral (VIS.) white adipose depots of 4-month-old female (a) and male (b) control and AT-ERαKO mutant siblings. Arrows indicate multilocular adipocytes present in the mutants. Scale bar=100 μm. (c–e) Relative mRNA levels of various brown adipocyte markers expressed in inguinal WAT (IWAT) of 4-month-old female (c) and male (d) or female interscapular classical BAT (e) of control and AT-ERαKO littermates were analysed (n≥6 each). (f) Inguinal adipose tissues from 4-month-old AT-ERαKO-GFP reporter mice were sectioned and stained for UCP1 (brown adipocyte protein) using immunohistochemistry. Arrows indicate UCP1+ multilocular cells. Scale bar=100 μm. (g,h) IWAT (g) and BAT (h) tissues from 4-month-old AT-ERαKO-GFP reporter female mice were sectioned and stained for GFP (adipose lineage sensitive marker, green), DAPI (nuclear stain, blue) and UCP1 (brown adipocyte protein, red). Arrow indicates UCP1+multilocular cells. Scale bar=50 μm for IWAT and 100 μm for BAT. Error bars indicate s.e.m. Statistical significance assessed by two-tailed Student’st-test, *P<0.05, **P<0.01. Figure 9: Progenitor deletion of ERα: brown adipose reprogramming. ( a , b ) H & E-stained histological sections of subcutaneous (SQ) and visceral (VIS.) white adipose depots of 4-month-old female ( a ) and male ( b ) control and AT-ERαKO mutant siblings. Arrows indicate multilocular adipocytes present in the mutants. Scale bar=100 μm. ( c – e ) Relative mRNA levels of various brown adipocyte markers expressed in inguinal WAT (IWAT) of 4-month-old female ( c ) and male ( d ) or female interscapular classical BAT ( e ) of control and AT-ERαKO littermates were analysed ( n ≥6 each). ( f ) Inguinal adipose tissues from 4-month-old AT-ERαKO-GFP reporter mice were sectioned and stained for UCP1 (brown adipocyte protein) using immunohistochemistry. Arrows indicate UCP1+ multilocular cells. Scale bar=100 μm. ( g , h ) IWAT ( g ) and BAT ( h ) tissues from 4-month-old AT-ERαKO-GFP reporter female mice were sectioned and stained for GFP (adipose lineage sensitive marker, green), DAPI (nuclear stain, blue) and UCP1 (brown adipocyte protein, red). Arrow indicates UCP1 + multilocular cells. Scale bar=50 μm for IWAT and 100 μm for BAT. Error bars indicate s.e.m. Statistical significance assessed by two-tailed Student’s t -test, * P <0.05, ** P <0.01. Full size image Brown adipocytes, in part due to UCP1 expression, ‘uncouples’ substrate oxidation from ATP production, generate heat rather than ATP [56] . The ensuing metabolic inefficiency can lead to increased energy expenditure and elevated body temperature [7] , [9] . To explore the possibility that the increased BAT observed in the AT-ERαKO mice might have functional consequences, we placed 4-month-old chow fed sibling control and mutant females in metabolic chambers and assessed a variety of relevant metabolic parameters such as food intake, energy expenditure, temperature and heat production, as we described [23] , [31] , [57] . Despite reduced body weight and adiposity, female mutants consumed about 1.5 times more food than controls ( Fig. 10a ). The mutants also had increased oxygen consumption (VO 2 ) and CO 2 production (VCO 2 ), indicating they have increased energy expenditure ( Fig. 10b ). Mutant respiratory quotient was increased during the light cycle when mice sleep ( Fig. 10c ), potentially secondary to a shift towards carbohydrate metabolism due to reduced adiposity [51] . These data indicate that the adipose lineage ERα-deficient mutants are hypermetabolic. 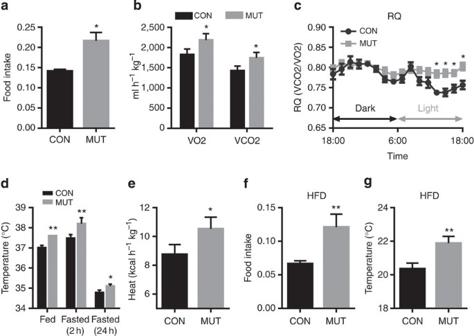Figure 10: AT-ERα mutants display a brown and a hypermetabolic phenotype. (a–c) Food intake (g per day per body weight) (a), oxygen consumption (VO2) and carbon dioxide production (VCO2) (b), and respiratory quotient (c, RQ) of 4-month-old female control and AT-ERαKO mice (n=6 each). (d) Body temperature (rectal probe) in fed, 2-h fasted (post-prandial) and 24-h fasted 4-month-old female control and AT-ERαKO mice. (e) Heat production of normal chow fed 4-month-old female control and AT-ERαKO siblings. (f–g) Food intake (f) and heat production (cage temperature) (g) of 4-month-old female control and AT-ERαKO mice fed 10 weeks of HFD (n=6 each). Error bars indicate s.e.m. Statistical significance assessed by two-tailed Student’st-test, *P<0.05, **P<0.01. Figure 10: AT-ERα mutants display a brown and a hypermetabolic phenotype. ( a – c ) Food intake (g per day per body weight) ( a ), oxygen consumption (VO 2 ) and carbon dioxide production (VCO 2 ) ( b ), and respiratory quotient ( c , RQ) of 4-month-old female control and AT-ERαKO mice ( n =6 each). ( d ) Body temperature (rectal probe) in fed, 2-h fasted (post-prandial) and 24-h fasted 4-month-old female control and AT-ERαKO mice. ( e ) Heat production of normal chow fed 4-month-old female control and AT-ERαKO siblings. ( f – g ) Food intake ( f ) and heat production (cage temperature) ( g ) of 4-month-old female control and AT-ERαKO mice fed 10 weeks of HFD ( n =6 each). Error bars indicate s.e.m. Statistical significance assessed by two-tailed Student’s t -test, * P <0.05, ** P <0.01. Full size image Oestrogen-deficient mammals have abnormal thermoregulation; elevated body temperature and hot flashes are prominent menopausal features [14] , [58] . To determine whether the adipose lineage might be involved in oestrogen-dependent temperature control, we examined body temperature in fed and fasted mice. The AT-ERαKO mutants displayed increased body temperature in both states ( Fig. 10d ). We also examined post-prandial thermogenesis, which can reflect BAT activity [59] ; this parameter was also increased in the mutants ( Fig. 10d ). Further, metabolic chamber analyses showed that heat production was similarly increased in AT-ERαKO mice ( Fig. 10e ). HFD-treated female mutants also displayed increased appetite and elevated heat production ( Fig. 10f,g ). Thus, loss of ERα signalling in adipose progenitor cells and throughout lineage specification leads to a brown phenotype, increased metabolic rate, elevated body temperature and increased appetite. Adipose tissues have a range of biological roles, spanning metabolism, lifespan control, behaviour modification, fertility and thermoregulation [60] , [61] , [62] . In turn, dietary, hormonal and environmental cues can remodel adipose tissue, can alter adipose tissue function and can regulate depot mass and adiposity [4] , [62] . These effects can be quite striking, for example, white adipose depots can be converted into energy burning BAT and body fat content can vary over 15-fold [63] . Such expansion can be detrimental; ample evidence exists that excess adipose tissue triggers a series of life-threatening sequela [64] . The remarkable ability of adipose tissue to expand, and the negative socio-economic-medical consequences linked to this change, highlights the urgent need to better understand how adipose tissue is formed and maintained, and to devise ways to regulate adiposity. Here we find that ERα signalling may be an excellent avenue; ERα controls adipose progenitor cell identity and fate decisions, determining entry into a white or brown adipose lineage or into smooth muscle fates. Further, mice with adipose lineage ERα mutation are lean, glucose sensitive, resist HFD and hypermetabolic, potentially secondary to changes of the adipose progenitor compartment. Adipose progenitor cells are essential to the development and maintenance of adipose tissues and may underlie aspects of adipose tissue plasticity [64] , [65] . Adipose progenitors appear to reside in a therapeutically accessible perivascular niche [34] , [65] . Genetic and pharmacological studies indicate that adipose progenitor cells can be manipulated in vivo and in clinically desirable manner [66] , [67] . Therefore, the control of adipose progenitor cells has emerged as a promising therapeutic strategy [66] , [67] , [68] . Here we find that oestrogen signalling regulates adipose progenitor cell function, in a manner that may be co-opted to manipulate the adipose lineage for clinically effective outcomes. Oestrogen regulates a range of physiological processes including various aspects of metabolism: fat mass, fat distribution, appetite, energy expenditure, temperature and glucose homeostasis [17] , [20] , [22] . The ability of oestrogen signalling to remodel fat depots and to alter distribution in a depot-specific manner is consistent with the notion that oestrogen may have direct effects on adipose progenitor cells [22] , [23] . Much of the metabolic control conferred by oestrogen appears to be transduced via ERα [21] , [26] . Many of these effects have been ascribed to roles of ERα in the CNS [23] . Here we find that several metabolic aspects of oestrogen appear linked to the roles of ERα within the adipose lineage per se . For example, surgical menopause (that is, OVX) altered adipose progenitor cell proliferation and progenitor cell number. Further, ERα has prominent expression in the adipose lineage, including the highest levels in progenitor cells that reside in a perivascular niche. To attempt to further investigate a potential cell autonomous role of oestrogen/ERα signalling in adipose progenitor cells, we generated a mouse model, AT-ERαKO, to delete ERα in adipose progenitor cells and throughout lineage specification. Notably, both female and male AT-ERαKO-mutant mice displayed several unexpected phenotypes that highlight ERα control of adipose progenitor cell function and developmental potential. Although whole-body, brain and mature adipocyte-specific ERα mutants and oestrogen-deficient mammals (for example, OVX) have increased adiposity [23] , [24] , [25] , [26] , the adipose lineage ERα deletion markedly reduced adiposity in subcutaneous and visceral depots. The phenotypic differences—AT-ERαKO mutants are lean, whereas whole-body, epiblast or mature adipocyte ERα mutants are obese—highlight the possibility that actions of ERα in other sites help determine final adipose morphology, mass and metabolic state; for example, in the CNS triggering increased food consumption or within adipocytes stimulating lipid accumulation. Consistent with that notion, HFD increased adipocyte formation and fat accumulation in AT-ERαKO mice. Further support for non-autonomous influences derives from our observation that ovariectomized mice exhibit accelerated adipose progenitor proliferation; a potential compensatory mechanism to replenish oestrogen-deprived progenitors. The AT-ERαKO depots have detectable aromatase expression, supporting the possibility that paracrine effects mediated by compensated local oestrogen production may also have such non-autonomous actions [69] . However, aromatase-deficient mice are obese rather than lean, as we observed in the AT-ERαKO mice that have lower aromatase levels [70] . Intriguingly, female AT-ERαKO mice display different magnitude of phenotypical effect on subcutaneous versus visceral fat depots, as lack of ERα has more detrimental outcome in the subcutaneous tissues as compared with visceral tissues, in accordance with higher expression of ERα in the subcutaneous fat. This observation should be taken into account based on the distinct metabolic features of these two types of fat depots: subcutaneous fat is known to be more metabolically favourable [2] . Utilizing the AdipoTrak murine model, we attempted to investigate the role of ERα in the adipose lineage; however, some aspects of the phenotype may be non-autonomous, mediated by PPARγ-knock-in-driver, as PPARγ exhibits a substantial metabolic function in other tissues, including the brain, muscle, endothelium and adipose-resident macrophages [35] , [36] , [37] , [38] . Still, several lines of evidence indicated that aspects of the reduced adipose phenotype observed in AT-ERαKO mice were secondary to actions of ERα signalling within adipose progenitors per se . For example, AT-ERαKO-mutant progenitors displayed blunted adipogenic differentiation in vivo , in organotypic settings and in cell culture, indicating a cell autonomous effect. The inhibited adipogenic potential of AT-ERαKO mutant progenitors was accompanied by increased adipose depot vascularity/angiogenesis that appeared secondary to altered adipose lineage specification. We also observed this hypervascular phenotype in epiblast-driven ERα-mutant mice, indicating that the effect is generalizable. Our data also indicate that the striking vasculogenic effects observed in the AT-ERαKO mice were secondary to an adipose progenitor cell fate change: ERα mutant adipose progenitors were reprogrammed into a vascular smooth muscle mural lineage. This adipogenic to vasculogenic fate change resonates with previous data showing oestrogen inhibits smooth muscle cell proliferation [41] , [42] , [43] , [44] , [45] . The smooth muscle fate transformation was accompanied by an activated angiogenic/vascular programme that we observed in vivo , in organotypic assays and in isolated progenitor cells. Our mechanistic studies indicated that the smooth muscle reprogramming was at least partially mediated by enhanced TGFβ signalling. For example, AT-ERαKO mutants had increased expression of TGFβ ligands and an activated TGFβ signalling cascade. Further, TGFβ-1 was sufficient to induce the adipogenic to mural fate change in cultured progenitors. Further, TGFβ signalling was required for the transformation; in necessity tests, a TGFβ inhibitor reversed the smooth muscle programme and rescued adipogenesis. The observed lineage change and blunted adipogenic differentiation appeared to confer significant and clinically desirable metabolic benefit: AT-ERαKO-mutant mice were lean, had increased glucose sensitivity and resisted untoward consequences of caloric excess. Oestrogen signalling also appeared to regulate another clinically relevant aspect of adipose progenitor cell potency, controlling a white versus brown adipogenic differentiation programme. For example, AT-ERαKO mutant white adipose depots had a surfeit of multilocular adipocytes that indicate the presence of brown-like energy burning adipocytes. Consistent with that notion, we found that the AT-ERαKO mutants had increased expression of a variety of BAT markers in both WAT and classical BAT. It is possible that the observed activated brown adipogenic potential was secondary to the increased vascular smooth muscle mural compartment; a recent report indicated that smooth muscle cells are endogenous induced brown adipocyte progenitors [71] . The white to brown lineage change appeared linked to functional changes in metabolism: AT-ERαKO mice were hypermetabolic, hyperphagic and hyperthermic. The elevated body temperature may reflect aspects of menopausal temperature abnormalities; if so, adipose progenitor ERα may be a potential therapeutic target for hot flashes and related issues. Adipose tissues play critical roles in metabolism and are at the core of a global ‘Diabesity’ epidemic. Yet, adipose tissues may harbour seeds for change; our ERα studies indicate that adipose progenitor cells may be tripotent in vivo . ERα signalling promotes white adipose progenitor cell identity and white lineage formation; ERα deficiency reprogrammes the cells into a smooth muscle or brown adipose differentiation programme. This can have significant physiological consequences; the AT-ERαKO female mice are lean, have increased energy expenditure, improved glucose sensitivity and resist HFD. Thus, adipose progenitor cells have significant in vivo plasticity and can form a variety of cell types depending on the relevant morphogenetic signalling context. These observations indicate that the development of selective oestrogen receptor modulation of adipose progenitor cells may be an appropriate strategy for obesity and diabetes, and possibly for vasomotor symptoms (hot flashes) characteristic of oestrogen deficiency. Animals The PPARγ-tTA, TRE-Cre, Sox2-Cre, floxed ERα, TRE-H2B-GFP, R26R-RFP and R26R-lacZ mice were maintained as described and used to generate controls, mutants and lineage reporter mouse lines [29] , [30] , [31] . AdipoTrak mice are defined as PPARγ-tTA; TRE-Cre; TRE-H2B-GFP. AT-ERαKO mutants are homozygous for ERα f/f allele, while controls are homozygous for ERα +/+ or lack TRE-Cre regardless of ERα alleles. The mice were housed in a temperature-controlled environment using a 12:12 light/dark cycle, and chow and water were provided ad libitum . The mice were fed either normal chow (4% fat, Harlan-Teklad, Madison, WI) or HFD (60%, Harlan Teklad). Fat content was measured using a minispec mq10 NMR Analyzer (Bruker). For glucose and insulin tolerance tests, 1.25 mg glucose or 1.5 mU Humalog (Lilly)/g mouse weight was injected intraperitoneally (IP) after a 5-h fast; blood glucose levels were measured at the indicated intervals [31] , [57] . BrdU was IP injected (100 mg kg −1 body mass) or provided in the drinking water (0.5 mg ml −1 in 1% sucrose). Sera insulin was measured by using an ELISA kit in the metabolic core. Veterinary care was provided by Division of Comparative Medicine. Animals were maintained under UT Southwestern Medical Center Animal Care and Use Committee guidelines according to current NIH guidelines under animal protocol 2010-0015. Adipose tissue fractionation In brief, SV cells were isolated from pooled white adipose depots, either subcutaneous (inguinal, interscapular) or visceral (perigonadal, retroperitoneal). The tissues were explanted and minced into fine pieces and then digested in adipocyte isolation buffer (100 mM HEPES pH7.4, 120 mM NaCl, 50 mM KCl, 5 mM glucose, 1 mM CaCl 2 , 1.5% BSA) containing 1 mg ml −1 collagenase at 37 °C with constant slow shaking (~120 r.p.m.) for 2–3 h. The suspension was then passed through a 200-μm mesh to remove undigested clumps and debris. The effluent was centrifuged at 500 g for 10 min, after which the floated adipocytes were collected from the top. The pellet was subjected to erythrocyte lysis buffer (8.3 g l −1 NH 4 Cl) for 5 min, washed in PBS and passed through 80 μm. Following another centrifugation, the resultant isolated SV cells were either cultured or subjected to FACS. Cell culture SV cells were cultured in DMEM with 10% FBS, 100 units per ml penicillin and 100 mg ml −1 streptomycin. TGFβ1 (10 ng ml −1 , PeproTech) was also added to one of the experiments. For induction, confluent wells were maintained in growth media supplemented with 1 mg ml −1 insulin, 3.5 μg ml −1 dexamethasone and 0.5 mM IBMX (all from Sigma) for 2–3 days and then only with insulin for about a week. Oil Red O staining was as described [72] . Metabolic chamber analyses Physical activity and energy expenditure were monitored using a combined indirect calorimetry system (TSE Systems GmbH, Bad Homburg, Germany). Mice were housed individually at room temperature (22 °C) under an alternating 12:12-h light-dark cycle. To avoid the possible confounding effects from diverged body weight and lean mass on energy expenditure [73] , we measured body weight, fat mass and lean mass before mice entered the metabolic chambers and normalized heat production values by lean mass. HFD-fed mice were acclimatized in the TSE metabolic chambers as described above. Heat production was continuously monitored for the 24-h fasting period and the following 24-h re-feeding period. Histology and immunohistochemistry Tissues were formalin-fixed and paraffin-embedded. Five to eight micron sections were cut and stained with haematoxylin and eosin. For immunohistochemistry, sections were deparaffinized, boiled in antigen-retrieval solution, treated with a rabbit anti-UCP1 antibody (1:200, Abcam #ab10983) and stained with Vectastain ABC KIT (Vector Laboratories) and DAB (ThermoScientific). Paraffin-embedded tissues were sectioned with a Microm HM 325 microtome. Immunofluorescence Immunofluorescence was performed on 5–8 μm cryostat sections of tissues freshly embedded in OCT as described [29] . The sections were fixed in 4% paraformaldehyde in PBS and then stained with rat anti-PECAM (1:200, BD Biosciences #557355), mouse anti-α smooth muscle actin (1:200, Abcam #ab7817), rabbit anti-phospho-JNK (1:200, Cell Signaling), rabbit anti-UCP1 (1:200, Abcam #ab10983) and rabbit anti-ERα (1:200, Abcam #ab2746) as described [29] . Secondary antibodies, used at a 1:500 dilution, included cy3 donkey anti-rabbit, cy3 donkey anti-mouse, cy3 donkey anti-rat, cy5 donkey anti-rat, cy5 donkey anti-rabbit, cy3 donkey anti-mouse were from Jackson ImmunoResearch. Immunostaining images were collected on a Zeiss LSM500 confocal microscope, an Olympus IX70 inverted microscope or an Olympus upright BX40 microscope. Direct GFP and RFP fluorescence for whole-adipose depots were imaged and photographed with a Zeiss Stemi SV11 microscope. Cryostat sectioning was performed with a Microm HM505 E cryostat. For BrdU staining, the cells, sections or tissues were fixed and washed in H 2 O, incubated with 1 N HCl at 37 °C for 45 min, washed in H 2 O, incubated in 0.1 M NaBO 4 for 10 min and subjected to immunohistochemistry. Ex vivo angiogenic potential Freshly collected adipose tissues were cut into ≈1-mm 3 pieces. The pieces were embedded in 35-mm glass bottom culture dishes (MatTek Corporation) containing 40 μl of growth factor-depleted Matrigel (BD Discovery Lab). Wells were filled with 200 μl of DMEM media supplemented with 10% of FBS and 1% Penicillin/Streptomycin, half of media was replaced every second day and angiogenic sprouts were analysed at days 7 and 14 in culture. Real-time PCR Total RNA was extracted using TRIzol (Invitrogen) from either mouse adipose tissue or SV cells, cDNA synthesis was performed using Superscript III reverse transcriptase (Invitrogen) as described [35] , [59] . Gene expression was analysed using Power SYBR Green PCR Master Mix with ABI 7500 Real-Time PCR System. qPCR values were normalized to β-actin or S18 expression. Primer sequences are presented in Supplementary Table 1 . Flow cytometry SV cells were isolated as above, washed, centrifuged at 800 g for 5 min and analysed with a FACScanto analyzer. Data analysis was performed using BD FACS Diva software. For SMA + , PECAM + and GFP + flow analysis, SV cells from either control or mutant mice were stained with a rabbit anti-αSMA antibody (1:200) and a rat anti-PECAM antibody (1:200) on ice for 30 min. Cells were then washed twice with the staining buffer and incubated with cy5 donkey anti-rabbit and cy3 donkey anti-rat secondary antibodies (1:500) for another 30 min on ice before flow cytometric analysis. BrdU detection of SV cells was performed with the APC BrdU Flow Cytometry Kit, according to the manufacturer’s instructions. Adipocyte nuclei were fixed in nuclei wash buffer, containing 4% formaldehyde before the BrdU detection and spun at 3,000 g . Statistical analyses Statistical significance assessed by two-tailed Student’s t -test. Error bars indicate s.e.m. How to cite this article: Lapid, K. et al. Oestrogen signalling in white adipose progenitor cells inhibits differentiation into brown adipose and smooth muscle cells. Nat. Commun. 5:5196 doi: 10.1038/ncomms6196 (2014).